Increasing water cycle extremes in California and in relation to ENSO cycle under global warming Since the winter of 2013–2014, California has experienced its most severe drought in recorded history, causing statewide water stress, severe economic loss and an extraordinary increase in wildfires. Identifying the effects of global warming on regional water cycle extremes, such as the ongoing drought in California, remains a challenge. Here we analyse large-ensemble and multi-model simulations that project the future of water cycle extremes in California as well as to understand those associations that pertain to changing climate oscillations under global warming. Both intense drought and excessive flooding are projected to increase by at least 50% towards the end of the twenty-first century; this projected increase in water cycle extremes is associated with a strengthened relation to El Niño and the Southern Oscillation (ENSO)—in particular, extreme El Niño and La Niña events that modulate California’s climate not only through its warm and cold phases but also its precursor patterns. As of mid-November 2014, the majority of the reservoirs in California were at extremely low levels: Lake Oroville, the second largest reservoir in California, lay at 26% of its full capacity, despite being at 90% in April 2013 ( http://cdec.water.ca.gov/ ). A drought state of emergency was declared in California in January 2014 ( http://gov.ca.gov/news.php?id=18379 ) in response to historic water shortfalls, as well as an increasing number of wildfires. The total statewide economic cost of the 2013–20114 drought is estimated at $2.2 billion, with a total loss of 17,100 jobs [1] . Given continuing drought conditions, a pressing question posed is whether the state of California will experience more frequent drought conditions in upcoming years. The effects of global warming on the regional climate include a hotter and drier climate [2] , [3] , as well as earlier snowmelt [4] , both of which exacerbate drought conditions. An understanding of the mechanisms that govern changes in extreme events at the regional scale is difficult, as they are likely caused by both anthropogenic CO 2 emissions and natural variability [5] . Many climate models participating in the Coupled Model Intercomparison Project Phase 5 (CMIP5) suggest a gradual increase in California’s precipitation in response to an increasing CO 2 concentration [6] , [7] , [8] . Globally, increasing CO 2 manifests in fewer occurrences of moderate rain but more light and heavy rain [9] . However, these changes in the mean state and characteristics cannot by themselves explain increasing drought severity as is the case for California or other similar extreme hydrological events. At face value, the CMIP5 projections of a wetter climate contradict the ‘hot and dry’ conditions conducive to increased droughts at the regional scale, as was recently pointed out as an argument for discounting a global warming connection in the 2013–2014 California drought [10] . Projected change in water cycle extremes in California Given the significance of extreme events within California with respect to climate change forcing, we analyse here multiple projections made by the Community Earth System Model version 1 (CESM1); this model has been shown to reasonably capture the variability of precipitation in California [5] , alongside multiple climate models that participated in the CMIP5. Under the RCP8.5 climate change scenario, CESM1 projects a gradual increase in California’s precipitation accompanied with increasing surface warming from 1990 through 2070 ( Fig. 1a and Supplementary Fig. 1 ); this is consistent with the CMIP5 ensemble [6] ( Fig. 2a ). A slight increase in precipitation occurs during boreal winter, yet temperature increases uniformly during all months ( Supplementary Fig. 2 ). We derive a metric of ‘water cycle extremes’, which is defined as the occurrence of both excessively wet and dry events per year in which the standardized precipitation index (SPI) exceeds ±2 in magnitude (see Methods section); this metric is designed to quantify the degree to which California experiences the alternation between extreme wet and extreme dry events. 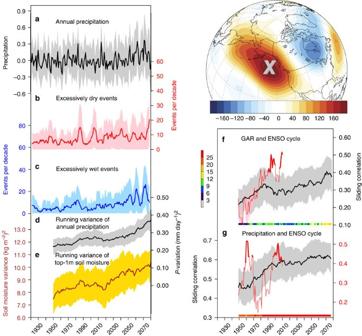Figure 1: Changing water cycle extremes in California simulated by CESM1. (a) Annual mean precipitation, (b) excessively dry events per year with 5-year running average (see text and Methods section), (c) excessively wet events per year with 5-year running average, (d) 30-year running variances of annual precipitation and (e) 30-year running variances of annual soil moisture in the top 1 m of soil layers averaged over California. Solid lines indicate a 30-member ensemble mean of CESM1, while shaded areas indicate model spread; roughly 50% of the ensemble members are within the shaded areas (see Methods section). The inset map atop (f) shows the November 2013–January 2014 geopotential height anomaly at 200 hPa depicting the GAR and the center location for the GAR index (cross). Right panels: the multivariate correlations between the Niño-3.4, Niño-3.4(Y+1) and (f) Gulf of Alaska Ridge (GAR) index and (g) annual precipitation averaged for water year in California, defined as October to September in the following year, within a running 30-year window during the NDJ season. The red line infis the multivariate correlation (r; see Methods section for formula) derived from the reanalysis data and that ingis from observed SST and precipitation (see Methods section). Note that theyaxis scale is different ingfor model (black; left) and for observation (red; right). Statistical significance of the multivariate correlations is given as a colour bar ing,fshowing the number of the ensemble members that are significant with 90% confidence based on the F-test. Similarly, thicker red lines represent the years with 90% significance. Figure 1b shows that the occurrence of excessively dry events in California increases considerably, and Fig. 1c indicates an even more pronounced increase in the occurrence of excessively wet events. These results indicate that future water cycle extremes will fluctuate more drastically between increasingly excessively wet and dry years. For instance, extreme dry event occurrence increases from about 5 over the period of 1930–1939 to about 10 over the period of 2070–2079 (that is, twofold), while extreme wet event occurrence increases from about 4 during 1930–1939 to roughly 15 during 2070–2079 (that is, roughly threefold). In essence, the rate of increase in extreme wet events is considerably higher than that of extreme dry events; this result is also consistent as realized from the multiple climate models in the CMIP5 ensemble ( Fig. 2b,c ). We note a difference between CMIP5 and CESM1 that the increase in excessively dry event frequency is larger than that for wet events in CMIP5. Moreover, 30-year running variances of both annual precipitation ( Fig. 1d for CESM1 and Fig. 2d for CMIP5 models) and the top 1-m soil moisture content ( Fig. 1e ) mirror the water cycle extremes index, that is, continually increasing towards the end of the twenty-first century. Observed rainfall also shows an increase in the 30-year running variance ( Supplementary Fig. 3 and Supplementary Note 1 ). Figure 1: Changing water cycle extremes in California simulated by CESM1. ( a ) Annual mean precipitation, ( b ) excessively dry events per year with 5-year running average (see text and Methods section), ( c ) excessively wet events per year with 5-year running average, ( d ) 30-year running variances of annual precipitation and ( e ) 30-year running variances of annual soil moisture in the top 1 m of soil layers averaged over California. Solid lines indicate a 30-member ensemble mean of CESM1, while shaded areas indicate model spread; roughly 50% of the ensemble members are within the shaded areas (see Methods section). The inset map atop ( f ) shows the November 2013–January 2014 geopotential height anomaly at 200 hPa depicting the GAR and the center location for the GAR index (cross). Right panels: the multivariate correlations between the Niño-3.4, Niño-3.4( Y+1 ) and ( f ) Gulf of Alaska Ridge (GAR) index and ( g ) annual precipitation averaged for water year in California, defined as October to September in the following year, within a running 30-year window during the NDJ season. The red line in f is the multivariate correlation ( r ; see Methods section for formula) derived from the reanalysis data and that in g is from observed SST and precipitation (see Methods section). Note that the y axis scale is different in g for model (black; left) and for observation (red; right). Statistical significance of the multivariate correlations is given as a colour bar in g , f showing the number of the ensemble members that are significant with 90% confidence based on the F-test. Similarly, thicker red lines represent the years with 90% significance. 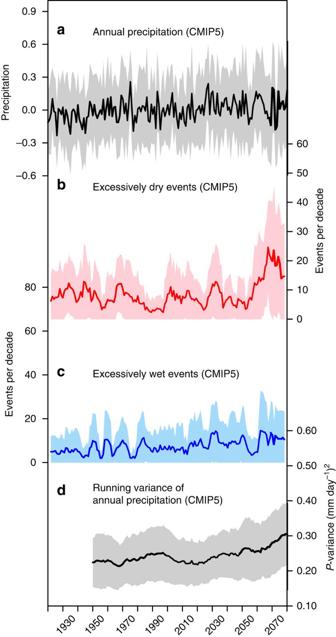Figure 2: Changing water cycle extremes in California simulated by CMIP5 models. (a) Annual mean precipitation, (b) excessively dry events per year with 5-year running average, (c) excessively wet events per year with 5-year running average, and (d) 30-year running variances of annual precipitation averaged over California from 25 climate models in CMIP5. Full size image Figure 2: Changing water cycle extremes in California simulated by CMIP5 models. ( a ) Annual mean precipitation, ( b ) excessively dry events per year with 5-year running average, ( c ) excessively wet events per year with 5-year running average, and ( d ) 30-year running variances of annual precipitation averaged over California from 25 climate models in CMIP5. Full size image Strengthened impact from El Niño Southern Oscillation cycle The role of climate variability in modulating water cycle extremes provides a key for anticipating the occurrence of extreme hydrological events. The El Niño Southern Oscillation (ENSO) has long been recognized as the prime climate modulator of precipitation and snowpack in California [11] , [12] , [13] . However, the winter of 2013–2014 was neither associated with an El Niño nor a La Niña event and yet, a record high-amplitude ridge developed and persisted over the Gulf of Alaska (referred to as the Gulf of Alaska Ridge (GAR)), blocking the majority of synoptic waves from impacting the West Coast [14] . The location of the GAR is shown in the inset of Fig. 1 . The consequential anomalous circulation pattern downwind, accompanied by a deep trough over eastern North America, is referred to as the dipole [5] (coined the ‘polar vortex’ by the media). The GAR’s persistence is not directly tied to ENSO but, instead, is correlated with a type of ENSO precursor [5] , [15] . Consequently, climate variability in California is modulated by the warm/cold phases of ENSO along with the transitions between them (that is, the ENSO precursor) formulating a complete cycle of ENSO. What is more important is to underscore the effects of increased greenhouse gases on the GAR’s high amplitude in the winter of 2013–2014 and the accompanying deep trough in eastern North America as highlighted in two recent studies [16] , [17] . Figure 1f shows the linear multivariate correlations between the Niño-3.4 index ( Y ), the Niño-3.4 index with 1 year lag ( Y+1 ), and the GAR index ( Y ; derived from the 200-hPa geopotential height; see Methods section) during the November–December–January (NDJ) timeframe; this is when the GAR–ENSO connection is most prominent in the beginning of the rainy season in California, following Wang et al [16] . Combination of Niño-3.4 ( Y ) and Niño-3.4 ( Y+1 ) represents an ENSO cycle as a whole including both its peak and precursor (see Methods section). Sliding correlations reveal a persistent increase in the association between the ENSO cycle and the GAR after 1995. A similar correlation analysis using reanalysis data (red line in Fig. 1f ) indicates an even more pronounced increase up to 2012; this echoes the observational increase in the correspondence between the ENSO cycle and California droughts after the 1960s [16] . It is of note that the CESM1 ensemble underestimates the level of increase in the ENSO–GAR correlation; this is not surprising since each of the 30 members featured different internal variations and the model may not accurately represent historical variations in other forcing agents such as aerosols [18] . However, Fig. 1g and Supplementary Fig. 4 show the association between simulated precipitation in California and the ENSO cycle in the NDJ season, and the correlations are in accordance with the ENSO–GAR correlations, despite its seemingly slower increase in the CMIP5 models than the CESM1 ensemble ( Supplementary Fig. 5-6 and Supplementary Note 2 ). Observational rainfall data set (red line in Fig. 1g ) exhibits large swings, which could be caused by the modulation of low frequency variability such as the Pacific Decadal Oscillation [12] , [19] ( Supplementary Fig. 3 and Supplementary Note 1 ). Taking everything into account, the results suggest a future of increased influence of the ENSO cycle on the North Pacific atmospheric circulation (including the GAR) and subsequent amplification in water cycle extremes over California [20] . In summary, an increase in water cycle extremes over California due to increased greenhouse gases is consistently and robustly projected by the multi-ensemble of the CESM1 and the multiple climate models in the CMIP5 ( Fig. 3 ). Both extreme wet/dry and moderate wet/dry events increase, accompanied by a reduction in those that are coined as ‘normal’. The result of an enhanced association between the precipitation probability and the ENSO cycle implies that the magnitude of ENSO itself may intensify in the future. Indeed, in contrast to previous finding of no change in ENSO amplitude and frequency due to greenhouse warming [21] , [22] , [23] , recent studies [24] , [25] that took non-linear ENSO physics into account have found that extreme El Niño and La Niña events are projected to increase in frequency (see Supplementary Figs. 7-9 and Supplementary Note 3 for a summary about change in extreme El Niño and La Niña events simulated by CESM1). Uncovered here is the robust relationship between an increase of the water cycle extremes over California and that of extreme El Niño and La Niña events; this was found in the majority of the coupled climate models and most of the ensembles ( Supplementary Fig. 10 ). Only three models in the CMIP5 ensemble and no CESM1 large-ensemble member exhibits a decrease in the number of extreme ENSO events, and only five CMIP5 models and two CESM1 ensemble members exhibit a decreasing number of water cycle extremes in California ( Supplementary Fig. 10 ). Nonetheless, atmospheric teleconnections associated with the ENSO cycle are more likely to intensify as a result of the Pacific warming [21] , [25] ; such inferences also apply with respect to the teleconnections associated with ENSO precursors [26] . 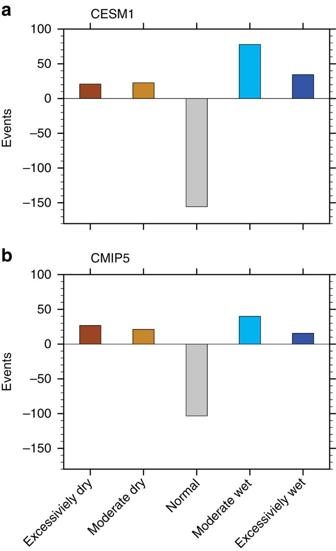Figure 3: Histogram of projected hydrological events change in California. Histogram of the extreme hydrological events change including excessively dry—defined as SPI<−2, moderate dry (−2≤SPI<−1), normal (−1≤SPI<1), moderate wet (1≤SPI<2) and excessively wet (SPI≥2) in three sub-regions of California with the CESM1 (a) and the CMIP5 models (b). Bootstrap method36is used to test statistical significance (see Methods section). Figure 3: Histogram of projected hydrological events change in California. Histogram of the extreme hydrological events change including excessively dry—defined as SPI<−2, moderate dry (−2≤SPI<−1), normal (−1≤SPI<1), moderate wet (1≤SPI<2) and excessively wet (SPI≥2) in three sub-regions of California with the CESM1 ( a ) and the CMIP5 models ( b ). Bootstrap method [36] is used to test statistical significance (see Methods section). Full size image Sensitivity experiment without oceanic feedbacks The increased association between ENSO teleconnections and California precipitation suggests an increase in the occurrence and intensity of water cycle extremes in California. Two sets of sensitivity experiments with a 1% CO 2 increase per year, one with oceanic feedbacks and the other without, are performed to further substantiate the connection between the ENSO and the intensification of water cycle extremes in California ( Fig. 4 ) and the role of the anthropogenic GHG. Without oceanic feedbacks in the global ocean (black lines), no significant change in precipitation variation is found, while, with a full dynamic ocean model, a consistent intensification occurs ( Fig. 1d , RCP8.5 scenario). 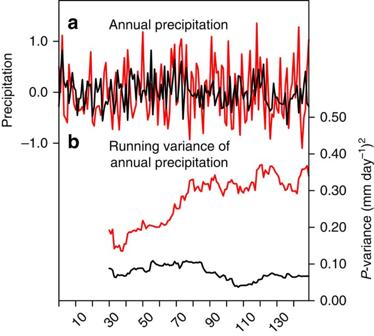Figure 4: A figure of sensitivity experiment. (a) Annual precipitation averaged over California from the 1% of CO2ramping experiment (red) and 1% CO2ramping experiment without global ocean feedback (black). (b) 30-year running variance of annual precipitation averaged over California. Figure 4: A figure of sensitivity experiment. ( a ) Annual precipitation averaged over California from the 1% of CO 2 ramping experiment (red) and 1% CO 2 ramping experiment without global ocean feedback (black). ( b ) 30-year running variance of annual precipitation averaged over California. Full size image Water cycle extremes in California, in terms of both drought and flood, will likely intensify despite the gradual increase of annual mean precipitation that can pose a new challenge in the management of already declining fresh water resources in the future [27] . The intensified water cycle extremes are linked to strengthened ENSO teleconnections, particularly extreme El Niño and La Niña events, which modulates California’s climate not only through its warm and cold phases, but also ENSO’s precursor patterns. Therefore, projections of drought must take into account the coupling within the ENSO cycle and ENSO-related teleconnections and above all, in the context of likely increasing extremes in non-linear fashion. The interplay of the climate dynamics associated with the extreme ENSO events throughout its whole life cycle described form a more complete representation of this particular climate system and, is an integral increment towards improvement in long-lead ENSO predictions [28] ; these ultimately drive more informed management practices that pertain to water resource management and supervision practices in California if not the Western US. CESM1 model output Thirty ensemble members were produced by the CESM1 with spatial resolution of 0.9 degrees longitude × 1.25 degrees latitude through the Large Ensemble Project [29] . The simulations cover two periods: (1) 1920–2005 with historical forcing, including greenhouse gases, aerosols, ozone, land use change, solar and volcanic activity, and (2) 2006–2080 with RCP8.5 forcing [30] . The ensemble spread of initial conditions is generated by the commonly used ‘round-off differences’ method [29] . CESM1 was used here partly because it well captures the ENSO cycle, ENSO precursors [31] , the associated teleconnections towards North America [16] , and as a result, precipitation variability in California. Detailed analysis on the performance of the CESM1 in terms of simulating the ENSO life cycle and rainfall over California is provided in Supplementary Figs 11–15 and Supplementary Note 4 for summary. CMIP5 model output 25 out of 38 coupled climate models ( Supplementary Tables 1 and 2 ) in CMIP5 are selected with a criteria previously used [24] , [25] , that is, the skewness of rainfall over Niño-3 region (5°S–5°N, 150°W–90°W) has to be larger than 1.0. Using satellite-based precipitation estimation [32] , the skewness of rainfall over Niño-3 region is 2.75 (ref. 25 ). Only the first ensemble member in each model is used here, though all the ensemble members of the CESM1 do produce the skewness larger than 2 ( Supplementary Table 2 bottom showing median, minimum, and maximum values). Number of excessively dry and wet events Numbers of excessively dry and wet events are determined using the SPI [33] , which is routinely used in drought monitoring and prediction by operational centres [34] , averaged over three sub-regions of California ( Supplementary Fig. 16 ). SPI is computed using monthly time series of accumulated precipitation, accumulated precipitation departure, and its percentile. Here we accumulate the months per year if SPI-12 values, SPI based on 12-month accumulated precipitation, exceed 2 (extremely wet) or −2 (extremely dry). In other words, one excessively dry event means at least one of the three sub-regions experienced an extremely dry month in a year and it can have values from 0 to 36. SPI-12 indicates a long-term drought on a 12-month time scale, which has more severe impacts on society and hydro-ecosystems. Reanalysis data Geopotential height and sea surface temperature (SST) from the twentieth century reanalysis project [35] were utilized. The advantage of the twentieth century reanalysis project is that it provides multiple ensemble members (56 total) to account for the uncertainty in the observation and data assimilation system, and this complements the evaluation of the large-ensemble CESM1 simulations. GAR index The GAR index was computed from the geopotential height at 200 hPa averaged within the domain (145°W–135°W, 45°N–55°N) over the North Pacific. This domain refers to the anomalous high center associated with the 2013–2014 NDJ anomaly, as shown in Fig. 1 inset map, and depicts the associated ridge-trough ‘dipole’ described in Wang et al [16] . Sensitivity experiment To isolate the effect of the oceanic feedback in the global ocean on water cycle extremes, we designed idealized sensitivity experiments: 1% CO 2 ramping experiment; The fully coupled CESM1 is integrated for 150 years from preindustrial conditions with CO 2 increasing by 1% per year. In this experiment, we expect to see the effects of anthropogenic warming on the global ocean and the water cycle extremes. 1% CO 2 ramping experiment without global ocean feedback, that is, sensitivity experiment; Same as the 1% CO 2 ramping experiment, except using prescribed SSTs instead of a dynamic ocean model. SSTs are linearly interpolated from the first and the last 10 years of the 1% CO 2 ramping experiment to have background warming in the ocean consistent with the imposed CO 2 forcing but no interannual variability. In other words, SST in the 1% CO 2 ramping experiment without global ocean feedback is computed as follows: where SST( y ) is the prescribed SST at year y with seasonal cycle, and is SST from the first experiment—1% CO 2 per year ramping experiment with dynamic ocean. Sea ice is constructed in the same manner. Contrasting these two experiments ( Fig. 4 ) indicates the importance of global oceanic feedbacks in amplifying water cycle extremes in a warming world. This experimental design removes oceanic feedbacks including not only increasing ENSO extremes but also change in SST variability in other part of the global ocean. Statistical significance test Changes in both excessively wet and dry events in California are statistically significant using the Bootstrap method [36] . The 18,000 monthly samples of SPI from the 30 members of CESM1 in the early period (1920–1969) are re-sampled randomly with the replacement to construct 10,000 realizations. The s.d. of the excessively wet and dry event frequency in the inter-realization is about 0.05/0.05 events per 1,500 years, much smaller than projected changes ( Fig. 3 ). Multivariate linear correlation Figure 1f,g , and Supplementary Figure 4 are based on the multivariate linear correlation ( r ). In case of dipole index and rainfall over California, the multivariate linear correlation with an ENSO cycle can be written as follows: Since the dipole signal could be strong either at the peak of ENSO or 1 year before ENSO, dipole index at any given year ( Y ) can be represented by both the contemporaneous Niño-3.4 index ( Y ) and the Niño-3.4 index 1 year later ( Y+1 ). The former represents dipole activity concurrently varying with the peak ENSO phases, while the latter depicts dipole intensity variation that occurs 1 year before the peak ENSO phases, signifying a ‘precursor’ pattern [5] . Combining both Niño-3.4 ( Y ) and Niño-3.4 ( Y+1 ) depicts an ENSO cycle as a whole. Correlation value ( r ) of dipole index with other indices is plotted in Fig. 1f,g , and Supplementary Fig. 4 . In a general linear model with n values ( y 1 , y 2 ,…, y n ) and corresponding modelled values based on the regression ( f 1 , f 2 ,…, f n ), r 2 is defined as while the residual (SS res ) and total sum of squares (SS tot ) are defined as where is the mean of the value. In this case, r is interpreted as the overall correlation of total variability in y i and the regressed value f i , and r 2 as the portion of total variability in y i accounted for by the linear regression. Running variance and correlation The sliding variance and correlation were computed for every 30-year span, for example, for the periods of 1920–1949, 1921–1950 and so on. This can be represented as the following equation: where is the average of A from Y −29 to Y . Running correlations are also computed in the similar manner: The GAR index The GAR index was computed as an area-averaged geopotential height at 200 mb over the North Pacific (145°W–135°W, 45°N–55°N). This domain refers to the anomalous high center associated with the 2013–2014 drought in California as shown in Fig. 1 (inset map) and explained in Wang et al [5] . In other words, an anomalously strong ridge (positive GAR index) is correlated with negative precipitation anomaly over California and the West coast of the United States in general. We choose the NDJ season for the GAR index because the NDJ season is when the GAR and the ENSO correlation are most prominent. This period is also the beginning of the wet season in California with abundant precipitation. Ensemble spread Throughout this work, a shaded area indicates the middle 50% of the spread of the ensemble members, calculated using z × s.d. In a normal distribution, the z value for 50% is 0.674490. How to cite this article: Yoon, J.-H. et al. Increasing water cycle extremes in California and relation to ENSO cycle under global warming. Nat. Commun. 6:8657 doi: 10.1038/ncomms9657 (2015).